The transcriptional repressor NKAP is required for the development of iNKT cells Invariant natural killer T cells have a distinct developmental pathway from conventional αβ T cells. Here we demonstrate that the transcriptional repressor NKAP is required for invariant natural killer T cell but not conventional T cell development. In CD4-cre NKAP conditional knockout mice, invariant natural killer T cell development is blocked at the double-positive stage. This cell-intrinsic block is not due to decreased survival or failure to rearrange the invariant Vα14-Jα18 T cell receptor-α chain, but is rescued by overexpression of a rec-Vα14-Jα18 transgene at the double-positive stage, thus defining a role for NKAP in selection into the invariant natural killer T cell lineage. Importantly, deletion of the NKAP-associated protein histone deacetylase 3 causes a similar block in the invariant natural killer T cell development, indicating that NKAP and histone deacetylase 3 functionally interact to control invariant natural killer T cell development. Invariant natural killer T (‘iNKT’) cells are a distinct, innate-type lineage of αβ T cells (reviewed in [1] , [2] ). In contrast to conventional αβ T cells that recognize peptide antigen presented on major histocompatibility complex (MHC) molecules, iNKT cells recognize glycolipids, such as α-GalCer and PBS-57, presented on the non-polymorphic MHC-like molecule CD1d. iNKT cells have limited T-cell receptor (TCR) diversity and express an invariant Vα14-Jα18 TCRα-chain combined with limited TCRβ-chains. iNKT cells comprise approximately 3% of mature thymocytes and splenic T cells, but account for ~30% of the liver lymphocyte population. Mature iNKT cells can be primed to produce significant quantities of multiple cytokines, including interferon-γ and interleukin-4, within minutes to hours after stimulation. iNKT cells follow a developmental pathway distinct from conventional T cells. At the CD4 + CD8 + double-positive (DP) stage, rearrangement and expression of the canonical Vα14-Jα18 TCR, and recognition of its cognate ligand, initiate selection into the iNKT cell lineage. At the TCRα locus, rearrangements are biased towards proximal V and J segments [3] . The Jα18 segment required for the iNKT invariant chain, however, is located distally. Therefore, the canonical Vα14-Jα18 iNKT TCRα usually occurs as a secondary rearrangement. Furthermore, mutations in genes that affect DP T cell survival cause a preferential defect in iNKT as compared with conventional αβ T cell development, as a shortened life span results in fewer secondary rearrangements [4] , [5] , [6] . Although conventional αβ T cells are selected on peptide/MHC expressed on thymic epithelial cells, iNKT cell development depends on positive selecting signals through recognition of glycolipid/CD1d complexes presented on DP T cells. In addition, stronger signals through the TCR are suggested to positively select DP T cells into iNKT cell lineage than conventional CD4 or CD8 T cells [7] . NKAP associates with DNA by chromatin immunoprecipitation, although this is likely indirect as NKAP lacks any previously characterized DNA-binding domains. NKAP associates with histone deacetylase 3 (Hdac3), and the Hdac3-binding domain is required for repression of transcription. NKAP also associates with CBF1-interacting repressor (CIR), which is part of the Notch corepressor complex, and NKAP has been demonstrated to be a negative regulator of Notch signalling. Conditional deletion of NKAP early in T cell development using Lck-cre led to a severe block in αβ T cell development at the DN3 to DP transition [8] . Deletion of NKAP at a later stage using CD4-cre, however, did not lead to any defects in the development or selection of conventional T cells in the thymus [9] . Here we show that deletion of NKAP with CD4-cre leads to an ablation of iNKT cell development. Furthermore, we show that deletion of NKAP-associated Hdac3 results in a similar disruption of iNKT cell development, implying functional interplay between these two factors that modulate gene expression. NKAP is required for iNKT cell development To determine whether NKAP had a role in iNKT cell development, we examined the thymus, spleen and liver for the presence of iNKT cells using CD1d tetramers loaded with the glycolipid PBS-57, or using unloaded CD1d tetramers as control. In CD4-cre NKAP conditional knockout (cKO) mice, although conventional T-cell development proceeded normally [9] there was a dramatic reduction of iNKT cells in the thymus ( Fig. 1a ). Similarly, iNKT cells were also missing from the spleen and liver of CD4-cre NKAP cKO mice ( Fig. 1b ). Therefore, the loss of NKAP leads to a severe block in iNKT cell development. 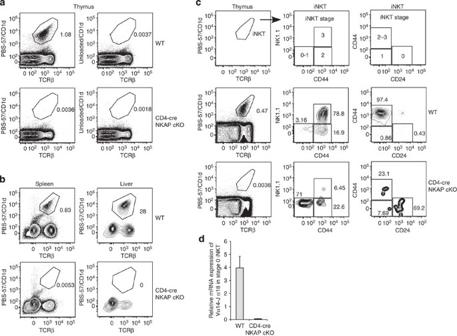Figure 1: NKAP is required for the development of iNKT cells. Lymphocytes from thymus (a), spleen and liver (b) were analysed for the presence of iNKT cells by flow cytometry using antibodies to TCRβ- and PBS-57-loaded CD1d tetramer to detect the presence of the canonical invariant TCR or empty CD1d tetramer alone without any associated glycolipid as a negative control. Data are representative of at least ten independent experiments. (c) Analysis of iNKT cell development from the earliest stage 0 (PBS-57/CD1d tetramer+TCRβ+CD24hiCD44−) to the latest stage 3 (PBS-57/CD1d tetramer+TCRβ+CD44+NK1.1+). Shown on the top is the gating strategy used in the analysis of iNKT cell development from WT thymocytes (middle row) and CD4-cre NKAP cKO thymocytes (bottom row). Data are representative of at least ten independent experiments. (d) Relative mRNA expression of the invariant Vα14-Jα18 TCR in stage 0 iNKT cells from WT and CD4-cre NKAP cKO mice. Stage 0 iNKT were isolated from CD4-cre NKAP cKO and WT littermates, by positive selection using PBS-57-loaded CD1d tetramer–PE/anti-PE-coated microbeads by MACS magnetic separation, followed by fluorescence-activated cell sorting for PBS-57/CD1d tetramer+TCR-β+CD24+NK1.1−stage 0 iNKT cells. cDNA was generated and examined for relative mRNA expression of the invariant Vα14-Jα18 TCR by qPCR. The data shown are the average expression of the invariant Vα14-Jα18 TCR from three WT and three CD4-cre NKAP cKO mice from three independent sorts. Data were normalized (=1) to the expression of the invariantVα14-Jα18TCR in one of the three WT mice. Error bars represent the s.e.m. Figure 1: NKAP is required for the development of iNKT cells. Lymphocytes from thymus ( a ), spleen and liver ( b ) were analysed for the presence of iNKT cells by flow cytometry using antibodies to TCRβ- and PBS-57-loaded CD1d tetramer to detect the presence of the canonical invariant TCR or empty CD1d tetramer alone without any associated glycolipid as a negative control. Data are representative of at least ten independent experiments. ( c ) Analysis of iNKT cell development from the earliest stage 0 (PBS-57/CD1d tetramer + TCRβ + CD24 hi CD44 − ) to the latest stage 3 (PBS-57/CD1d tetramer + TCRβ + CD44 + NK1.1 + ). Shown on the top is the gating strategy used in the analysis of iNKT cell development from WT thymocytes (middle row) and CD4-cre NKAP cKO thymocytes (bottom row). Data are representative of at least ten independent experiments. ( d ) Relative mRNA expression of the invariant Vα14-Jα18 TCR in stage 0 iNKT cells from WT and CD4-cre NKAP cKO mice. Stage 0 iNKT were isolated from CD4-cre NKAP cKO and WT littermates, by positive selection using PBS-57-loaded CD1d tetramer–PE/anti-PE-coated microbeads by MACS magnetic separation, followed by fluorescence-activated cell sorting for PBS-57/CD1d tetramer + TCR-β + CD24 + NK1.1 − stage 0 iNKT cells. cDNA was generated and examined for relative mRNA expression of the invariant Vα14-Jα18 TCR by qPCR. The data shown are the average expression of the invariant Vα14-Jα18 TCR from three WT and three CD4-cre NKAP cKO mice from three independent sorts. Data were normalized (=1) to the expression of the invariant Vα14-Jα18 TCR in one of the three WT mice. Error bars represent the s.e.m. Full size image iNKT cell development is blocked at the DP stage As iNKT cells develop, they proceed from the DP stage through four stages defined by cell-surface expression of CD24, CD44 and NK1.1: cells progress from stage 0 (CD24 hi CD44 − NK1.1 − ) to stage 1 (CD24 −/lo CD44 −/lo NK1.1 − ), then to stage 2 (CD24 − CD44 + NK1.1 − ) and finally to stage 3 (CD24 − CD44 + NK1.1 + ), as shown schematically in Fig. 1c . Using flow cytometry, we examined the various stages of iNKT cell development in CD4-cre NKAP cKO mice ( Fig. 1c ). In contrast to wild-type (WT) mice, the few tetramer + thymocytes in CD4-cre NKAP cKO mice expressed CD24, indicative of stage 0 iNKTs. However, these cells did not express the iNKT canonical Vα14-Jα18 TCRα chain, and thus are not stage 0 iNKT ( Fig. 1d ) [10] , [11] , [12] . Therefore, iNKT cell development in CD4-cre NKAP cKO mice is blocked at the DP stage. The block in iNKT cell development is cell-intrinsic The development of iNKT cells depends on positive selecting signals through glycolipids presented on DP T cells by the MHC class I-like molecule CD1d, as well as homotypic interactions through the SLAM family receptors Slamf1 (CD150) and Slamf6 (Ly108) [13] . To exclude the possibility that the block in iNKT development was due to lack of expression of any of these proteins in DP T cells, expression of CD1d, Slamf1 and Slamf6 was examined in WT and CD4-cre NKAP cKO mice. As shown in Fig. 2a , CD4 expression was equivalent in WT and CD4-cre NKAP cKO DP T cells. CD1d expression was decreased ~33% in CD4-cre NKAP cKO DP T cells as compared with WT. This change was unlikely to be the cause of the loss of iNKT cell development, as CD1d heterozygous mice express approximately half the amount of CD1d on the cell surface as WT B6 mice, but exhibit normal iNKT cell development [14] . Expression of Slamf1 and Slamf6 were slightly elevated (~30%) in CD4-cre NKAP cKO DP T cells as compared with WT. Therefore, the block in iNKT cell development in the absence of NKAP is not due to loss of expression of CD1d, Slamf1 or Slamf6. The failure in iNKT cell development could be due to an inability of NKAP-deficient cells to present endogenous glycolipids in CD1d. To determine if the block in iNKT cell development in CD4-cre NKAP cKO mice was cell-intrinsic, mixed bone marrow stem cell chimeras were generated. Bone marrow from CD4-cre NKAP cKO (CD45.2) mice and congenic B6.SJL (CD45.1) mice was used to reconstitute lethally irradiated B6.SJL recipients. Although thymocytes derived from both types of donor cells were observed, only WT B6.SJL-derived thymocytes, and not CD4-cre NKAP cKO thymocytes, developed into iNKT cells ( Fig. 2b ). Thus, the early block in iNKT cell development in CD4-cre NKAP cKO mice is cell-intrinsic. Furthermore, these data confirm that NKAP-deficient DP thymocytes cannot be selected into the iNKT cell lineage even in the presence of WT DP T cells. To understand the nature of the developmental defect, DP thymocytes from WT and CD4-cre NKAP cKO mice were examined by quantitative PCR (qPCR) for expression of genes necessary for iNKT cell development, including SAP [15] , [16] , [17] , Egr2 (ref. 18 ), Fyn [19] , [20] , c-Myc [21] , [22] , c-Myb [4] , Runx1 (ref. 6 )/ CBFβ , T-bet [23] and HEB [5] . However, all of these genes were expressed at similar levels (less than twofold difference in expression) in DP thymocytes from WT and CD4-cre NKAP cKO mice ( Fig. 2c ). Hence, the loss of NKAP does not alter the expression of many genes previously demonstrated to be required for iNKT cell development. 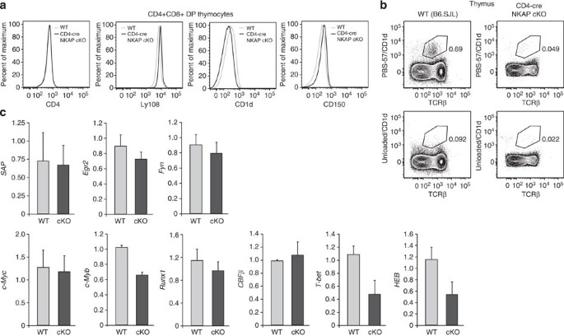Figure 2: Cell autonomous requirement for NKAP in iNKT cell development. (a) Expression of CD4, Ly108, CD1d and CD150 in DP thymocytes from CD4-cre NKAP cKO mice and WT littermate controls was examined using flow cytometry. The grey lines represent expression in WT DP thymocytes and the black lines represent expression in CD4-cre NKAP cKO DP thymocytes as denoted in the figure. Data are representative of at least two independent experiments. (b) Mixed stem cell chimeras were generated using equal proportions of bone marrow from WT B6.SJL congenic mice (CD45.1+) and CD4-cre NKAP cKO mice (CD45.2+), to reconstitute lethally irradiated B6.SJL recipients. Ten weeks later, thymocytes were examined for the development of iNKT cells (as inFig. 1) using the CD45.1 allelic marker to distinguish the contribution from each genotype. Results shown are representative of three mixed stem cell chimeras. (c) Expression of genes required for iNKT cell development. cDNA from fluorescence-activated cell-sorted DP thymocytes from CD4-cre NKAP cKO and WT littermates was examined for expression ofSAP,Egr2,Fyn,c-Myc,c-Myb,Runx1,CBFβ,T-betandHEB. Data shown are the average from two WT and two CD4-cre NKAP cKO mice from independent sorts. Data are normalized to the relative expression in one of the WT mice (=1). Error bars represent s.e.m. Figure 2: Cell autonomous requirement for NKAP in iNKT cell development. ( a ) Expression of CD4, Ly108, CD1d and CD150 in DP thymocytes from CD4-cre NKAP cKO mice and WT littermate controls was examined using flow cytometry. The grey lines represent expression in WT DP thymocytes and the black lines represent expression in CD4-cre NKAP cKO DP thymocytes as denoted in the figure. Data are representative of at least two independent experiments. ( b ) Mixed stem cell chimeras were generated using equal proportions of bone marrow from WT B6.SJL congenic mice (CD45.1 + ) and CD4-cre NKAP cKO mice (CD45.2 + ), to reconstitute lethally irradiated B6.SJL recipients. Ten weeks later, thymocytes were examined for the development of iNKT cells (as in Fig. 1 ) using the CD45.1 allelic marker to distinguish the contribution from each genotype. Results shown are representative of three mixed stem cell chimeras. ( c ) Expression of genes required for iNKT cell development. cDNA from fluorescence-activated cell-sorted DP thymocytes from CD4-cre NKAP cKO and WT littermates was examined for expression of SAP , Egr2 , Fyn , c-Myc , c-Myb , Runx1 , CBFβ , T-bet and HEB . Data shown are the average from two WT and two CD4-cre NKAP cKO mice from independent sorts. Data are normalized to the relative expression in one of the WT mice (=1). Error bars represent s.e.m. Full size image The block in development is not due to decreased DP survival The rearrangement of the canonical Vα14-Jα18 TCR chain is usually a secondary rearrangement, as the Jα18 gene segment is located distally. Mice with mutations that effect DP T cell survival have a preferential defect in iNKT as compared with conventional αβ T cell development, as a shortened life span results in fewer secondary rearrangements. iNKT cell development can be partially rescued in cases of decreased DP survival by overexpression of Bcl-2 or Bcl-x [4] , [5] , [6] . Thus, we examined whether decreased survival of DP thymocytes was the cause for the lack of iNKT cells in CD4-cre NKAP cKO mice. Using flow cytometry, we observed similar expression of Bcl-2, Nur77 and Annexin V in DP thymocytes from WT and CD4-cre NKAP cKO mice ( Fig. 3a ). By qPCR, mRNA transcript levels of Bcl-2, Bcl-x, Mcl-1 and Nur77 were similar in DP thymocytes of WT and CD4-cre NKAP cKO mice ( Fig. 3b ). We also generated Bcl-xL transgenic/CD4-cre NKAP cKO and Bcl-2 transgenic/CD4-cre NKAP cKO mice. However, overexpression of either Bcl-xL or Bcl-2 did not rescue iNKT cell development in these mice, as iNKT cells were not detected in the thymus ( Fig. 3c ), spleen and liver ( Supplementary Fig. S1 ). Furthermore, if loss of NKAP led to decreased survival we would expect to have seen a decrease in relative chimerism in DP and semimature CD4 single-positive (SP) thymocytes derived from CD4-cre NKAP cKO progenitors in mixed radiation chimeras ( Fig. 2b ). However, there was no difference in relative chimerism of DP and semimature CD4 SP population of CD4-cre NKAP-deficient thymocytes as compared with WT controls ( Fig. 3d ). Therefore, the early block in iNKT cell development in CD4-cre NKAP cKO mice is not due to decreased survival of DP thymocytes. 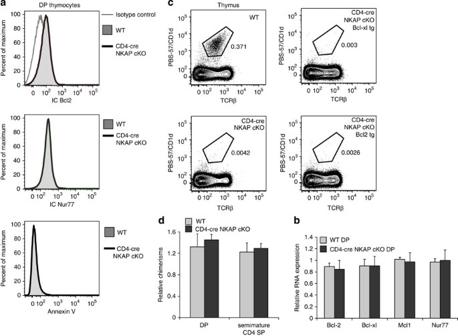Figure 3: The block in iNKT cell development is not because of decreased survival of DP thymocytes. (a)The expression of Bcl-2 (intracellular), Nur77 (intracellular) and Annexin V stain in DP thymocytes from WT and CD4-cre NKAP cKO mice was examined using flow cytometry. Data are representative of four independent experiments. (b)The relative RNA transcript levels of Bcl-2, Bcl-xL, Mcl-1 and Nur77 in sorted DP thymocytes was examined using qPCR. Differences in the relative expression of Bcl-2, Bcl-xL, Mcl-1 and Nur77 in DP thymocytes are not statistically significant between WT and CD4-cre NKAP cKO mice as calculated by Student’st-test. Data shown are the average from six WT and six CD4-cre NKAP cKO mice from three independent sorts. Data are normalized to the relative expression in one of the WT mice (=1). Error bars represent s.e.m. (c) The presence of iNKT cells in the thymus from WT, CD4-cre NKAP cKO, Bcl-2 transgenic/CD4-cre NKAP cKO and Bcl-xL transgenic/CD4-cre NKAP cKO mice was examined as inFig. 1. Data are representative of at least two mice per group from at least two independent experiments. (d) The relative chimerism of WT versus CD4-cre NKAP cKO bone marrow for DP and semimature CD4 SP T-cell population was examined from mixed bone marrow experiment as described in Fig.2. Data are representative of six control and six CD4-cre NKAP cKO mixed chimeras. Figure 3: The block in iNKT cell development is not because of decreased survival of DP thymocytes. ( a )The expression of Bcl-2 (intracellular), Nur77 (intracellular) and Annexin V stain in DP thymocytes from WT and CD4-cre NKAP cKO mice was examined using flow cytometry. Data are representative of four independent experiments. ( b )The relative RNA transcript levels of Bcl-2, Bcl-xL, Mcl-1 and Nur77 in sorted DP thymocytes was examined using qPCR. Differences in the relative expression of Bcl-2, Bcl-xL, Mcl-1 and Nur77 in DP thymocytes are not statistically significant between WT and CD4-cre NKAP cKO mice as calculated by Student’s t -test. Data shown are the average from six WT and six CD4-cre NKAP cKO mice from three independent sorts. Data are normalized to the relative expression in one of the WT mice (=1). Error bars represent s.e.m. ( c ) The presence of iNKT cells in the thymus from WT, CD4-cre NKAP cKO, Bcl-2 transgenic/CD4-cre NKAP cKO and Bcl-xL transgenic/CD4-cre NKAP cKO mice was examined as in Fig. 1 . Data are representative of at least two mice per group from at least two independent experiments. ( d ) The relative chimerism of WT versus CD4-cre NKAP cKO bone marrow for DP and semimature CD4 SP T-cell population was examined from mixed bone marrow experiment as described in Fig. 2 . Data are representative of six control and six CD4-cre NKAP cKO mixed chimeras. Full size image Recombination of iNKT TCRα is not altered by loss of NKAP Next, we examined whether loss of NKAP altered the recombination and expression of the canonical Vα14-Jα18 TCRα chain. One of the direct targets of NKAP is Skp2, a component of the E3 ubiquitin ligase Skp2-SCF [8] . Skp2-SCF regulates Rag2 protein expression during cell cycle, binding phosphorylated Rag2 and targeting it for degradation to prevent Rag-mediated recombination outside of the G1 cell cycle phase [24] . Skp2 deficiency is associated with persistence of Rag activity throughout the cell cycle [24] . As the loss of NKAP at the DP stage may lead to overexpression of Skp2, we considered the possibility that this could suppress distal rearrangements, including Vα14-Jα18, through enhanced degradation of Rag2. To test this, we crossed our CD4-cre NKAP cKO mice with Rag2-T490A knock-in mice, which have a mutation in the phosphorylation site required for the periodic destruction mediated by Skp2-SCF [24] . However, iNKT cell development remained blocked in CD4-cre NKAP cKO/Rag2-T490A mice ( Fig. 4a ), indicating that an increase in Skp2-SCF-mediated Rag2 ubiquitination is not responsible for the failure to generate iNKT cells. 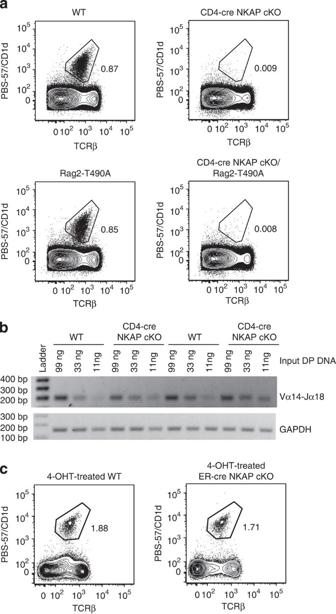Figure 4: The block in development is not because of failure to rearrange the Vα14-Jα18 TCRα chain. (a) The presence of iNKT cells in WT, CD4-cre NKAP cKO, Rag2(T490A) and CD4-cre NKAP cKO/Rag2(T490A) mice was examined using flow cytometry. Analysis was done as described inFig. 1. Data are representative of three independent experiments. (b) Vα14-Jα18 recombination was examined by semi-qPCR by serial dilution (99, 33 or 11 ng per PCR reaction) of genomic DNA from DP thymocytes from two WT and two CD4-cre NKAP cKO mice from independent sorts. Glyceraldehyde 3-phosphate dehydrogenase (GAPDH) was examined as a control. (c) The expression of invariant Vα14-Jα18 TCR of iNKT cells in 4-OHT-treated WT and ER-cre NKAP cKO mice was measured by the presence of PBS-57-CD1d-loaded tetramer stain using flow cytometry. Data are representative from four mice in each group. Figure 4: The block in development is not because of failure to rearrange the Vα14-Jα18 TCRα chain. ( a ) The presence of iNKT cells in WT, CD4-cre NKAP cKO, Rag2(T490A) and CD4-cre NKAP cKO/Rag2(T490A) mice was examined using flow cytometry. Analysis was done as described in Fig. 1 . Data are representative of three independent experiments. ( b ) Vα14-Jα18 recombination was examined by semi-qPCR by serial dilution (99, 33 or 11 ng per PCR reaction) of genomic DNA from DP thymocytes from two WT and two CD4-cre NKAP cKO mice from independent sorts. Glyceraldehyde 3-phosphate dehydrogenase (GAPDH) was examined as a control. ( c ) The expression of invariant Vα14-Jα18 TCR of iNKT cells in 4-OHT-treated WT and ER-cre NKAP cKO mice was measured by the presence of PBS-57-CD1d-loaded tetramer stain using flow cytometry. Data are representative from four mice in each group. Full size image To directly examine recombination of the canonical Vα14-Jα18 TCRα chain, DP thymocytes from CD4-cre NKAP cKO and WT mice were sorted. DNA rearrangement of Vα14-Jα18 was examined by semi-qPCR ( Fig. 4b ). Rearrangement of the invariant Vα14-Jα18 chain was similar between NKAP-deficient and WT thymocytes, demonstrating that the loss of NKAP does not result in a failure to recombine Vα14 with Jα18, to generate the canonical iNKT TCRα chain. Hence, the lack of iNKT cells in CD4-cre NKAP cKO mice is not due to a failure in rearrangement of the canonical Vα14-Jα18 TCRα chain. The loss of NKAP in DP thymocytes could also affect the expression level of the iNKT cell receptor; hence, we assessed the level of Vα14-Jα18 TCR expression in mature iNKT cell after loss of NKAP. Using ER-cre NKAP cKO mice, we induced NKAP deletion in vivo by 4-hydroxy-tamoxifen (4-OHT) and analysed the mean fluorescence intensity of iNKT TCR by tetramer staining with a PBS-57-loaded CD1d tetramer. As shown in Fig. 4c , there was no change in the expression of Vα14-Jα18 TCR in 4-OHT-treated ER-cre NKAP cKO as compared with 4-OHT-treated WT mice. Thus, deletion of NKAP does not alter expression of the TCR on iNKT cells. Overexpression of Vα14-Jα18 TCR rescues iNKT development As NKAP deficiency did not alter DP survival, Vα14-Jα18 rearrangement or iNKT TCR expression, another possibility is that NKAP functions in positive selection of DP thymocytes into the iNKT cell lineage. Stronger TCR signals are needed to positively select DP thymocytes into the iNKT lineage than conventional T cells [7] . Therefore, transgenic overexpression of Vα14-Jα18 may rescue iNKT cell development in CD4-cre NKAP cKO mice. However, although TCR expression normally does not appear at the cell surface until the DP stage, many TCR transgenes are expressed at the double-negative (DN) stage [25] . This is a significant complication, as premature expression of a rearranged TCR may allow for selection before conditional deletion at the DP stage using CD4-cre. Therefore, a new transgenic line in which expression of Vα14-Jα18 was delayed until the DP stage was needed. To restrict the expression of the transgene, the Vα14-Jα18 TCR chain was inserted into a modified pTαCass transgene vector with a reconstituted complete TCRα locus control region (LCR), as was previously described for the generation of ‘rec-HY’ transgenics [26] . This vector contains recombination signal sequences (RSS) and a 5-kb stuffer fragment inserted into the coding sequence after the initiating methionine, thus preventing expression of the transgene until the stuffer fragment is removed by RAG-mediated recombination. Using this system to express the HY TCRα chain in rec-HY mice, the timing and regulation of expression of the HY TCRα chain mirrors that of endogenous TCRα [26] . This system was used here to generate ‘rec-Vα14’ mice. Flow cytometry confirmed that the rec-Vα14 transgene is not expressed earlier than the endogenous iNKT TCR ( Supplementary Fig. S2 ). As shown in Fig. 5a , when crossed to CD4-cre NKAP cKO mice, expression of rec-Vα14 rescued development of iNKT cells in the thymus, and restored iNKT cells in the periphery ( Fig. 5a ). We examined the expression of the invariant Vα14-Jα18 TCR in WT, rec-Vα14 transgenic mice and rec-Vα14/CD4-cre NKAP cKO mice by measuring the mean fluorescence intensity of a CD1d-PBS-57-loaded tetramer stain using flow cytometry. There was ~20% increase in the expression of rec-Vα14-Jα18 TCRα chain in rec-Vα14 trangenic and rec-Vα14/CD4-cre NKAP cKO mice than that in the endogenous Vα14-Jα18 TCR of WT mice ( P -value<0.01 and P -value<0.001, respectively; Fig. 5b ). We also examined the absolute number of various stages of iNKT cells in the WT, rec-Vα14 and rec-Vα14/CD4-cre NKAP cKO mice. We observed a statistically significant increase in the number of immature stage 0, 1 and 2 (NK1.1 − ) iNKT cells in the rec-Vα14 and rec-Vα14/CD4-cre NKAP cKO mice as compared with WT mice ( Fig. 5c ), as may be expected due to increased expression of this transgene. However, there was no statistically significant change in the absolute number of mature stage-3 iNKT cells in the WT, rec-Vα14 and rec-Vα14/CD4-cre NKAP cKO mice. Thus, ectopic overexpression of the Vα14-Jα18 TCRα chain rescues iNKT cell development in the absence of NKAP. 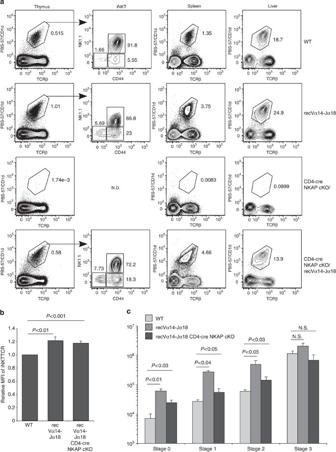Figure 5: Transgenic expression of invariant rec-Vα14-Jα18 TCRα chain rescues iNKT cell development. (a)The presence of iNKT cells in the thymus, liver and spleen from WT, CD4-cre NKAP cKO, recVα14-Jα18 TCR transgenic and CD4-cre NKAP cKO/recVα14-Jα18 TCR mice was examined as inFig. 1. Data are representative of at least four mice per group from three independent experiments. (b) The expression of invariant Vα14-Jα18 iNKT TCR from WT to recVα14 transgenic and WT to CD4-cre NKAP cKO/recVα14-Jα18 TCR transgenic mice was measured by the mean fluorescence intensity (MFI) of PBS-57-CD1d-loaded tetramer using flow cytometry. The difference in relative MFI is statistically significant using Student’st-test (P<0.01 andP<0.001, respectively). The relative MFI is mean from seven WT, nine recVα14-Jα18 TCR transgenic and six CD4-cre NKAP cKO/recVα14-Jα18 TCR transgenics mice from six independent experiments. (c) Absolute number of stages 0, 1, 2 and 3 iNKT cells in WT, recVα14-Jα18 TCR transgenic and CD4-cre NKAP cKO/recVα14-Jα18 TCR transgenics was calculated. The absolute number is the mean of four WT, six recVα14-Jα18 TCR transgenic and six CD4-cre NKAP cKO/recVα14-Jα18 TCR transgenic mice from three independent experiments. The differences in absolute numbers of immature stage 0, 1 and 2 iNKT cells from WT, recVα14-Jα18 TCR transgenic and CD4-cre NKAP cKO/recVα14-Jα18 TCR transgenics is statistically significant, using Student’st-test as denoted in the figure, whereas there are no differences in the absolute number of mature stage 3 iNKT cells (N.S., not significant). Figure 5: Transgenic expression of invariant rec-Vα14-Jα18 TCRα chain rescues iNKT cell development. ( a )The presence of iNKT cells in the thymus, liver and spleen from WT, CD4-cre NKAP cKO, recVα14-Jα18 TCR transgenic and CD4-cre NKAP cKO/recVα14-Jα18 TCR mice was examined as in Fig. 1 . Data are representative of at least four mice per group from three independent experiments. ( b ) The expression of invariant Vα14-Jα18 iNKT TCR from WT to recVα14 transgenic and WT to CD4-cre NKAP cKO/recVα14-Jα18 TCR transgenic mice was measured by the mean fluorescence intensity (MFI) of PBS-57-CD1d-loaded tetramer using flow cytometry. The difference in relative MFI is statistically significant using Student’s t -test ( P <0.01 and P <0.001, respectively). The relative MFI is mean from seven WT, nine recVα14-Jα18 TCR transgenic and six CD4-cre NKAP cKO/recVα14-Jα18 TCR transgenics mice from six independent experiments. ( c ) Absolute number of stages 0, 1, 2 and 3 iNKT cells in WT, recVα14-Jα18 TCR transgenic and CD4-cre NKAP cKO/recVα14-Jα18 TCR transgenics was calculated. The absolute number is the mean of four WT, six recVα14-Jα18 TCR transgenic and six CD4-cre NKAP cKO/recVα14-Jα18 TCR transgenic mice from three independent experiments. The differences in absolute numbers of immature stage 0, 1 and 2 iNKT cells from WT, recVα14-Jα18 TCR transgenic and CD4-cre NKAP cKO/recVα14-Jα18 TCR transgenics is statistically significant, using Student’s t -test as denoted in the figure, whereas there are no differences in the absolute number of mature stage 3 iNKT cells (N.S., not significant). Full size image The block in iNKT development is not due to Notch activation Previously, we demonstrated that NKAP is a transcriptional repressor and a component of the Notch corepressor complex. NKAP deletion during early T-cell development using Lck-cre led to an increase of 8- to 20-fold in the expression of the Notch target genes Deltex , CD25 and Hes1 in DP T cells [8] . Interestingly, recent evidence suggests that suppression of Notch signalling may be required for iNKT development to proceed. Embryonic stem cells can differentiate in culture into early CD24 hi CD44 lo iNKT cells [27] , when cultured on the well-characterized OP9/Dll1 system [28] . However, for iNKT maturation to proceed, early (stage 0) CD24 hi CD44 lo iNKT cells had to be transferred to OP9 stromal cells that lacked Dll1. One interpretation of these data are that Notch signalling must be downregulated for iNKT development to proceed [27] . As NKAP is a negative regulator of Notch signalling, one possibility was that the lack of iNKT cells in the CD4-cre NKAP cKO mouse results from constitutive activation of the Notch target genes. To test this, we examined iNKT cell development in CD4-cre NKAP cKO mice that also lacked RBP-Jκ [29] , the transcription factor through which cleaved intracellular Notch activates transcription. As shown in Fig. 6 , iNKT development was normal in CD4-cre RBP-Jκ cKO mice, demonstrating that Notch signalling is not necessary for the development of iNKT cells. However, iNKT cell development was still abrogated in CD4-cre NKAP cKO/RBP-Jκ cKO mice, demonstrating that the block in iNKT cell development in CD4-cre NKAP cKO mice is independent of the role of NKAP as a negative regulator of Notch signalling. 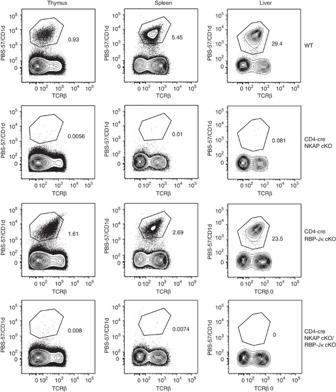Figure 6: The block in iNKT cell development due to loss of NKAP is independent of Notch activation. The presence of iNKT cells in the thymus, liver and spleen from WT, CD4-cre NKAP cKO, CD4-cre RBP-Jκ cKO and CD4-cre NKAP cKO/ RBP-Jκ cKO mice were examined as inFig. 1. Data are representative of four independent experiments. Figure 6: The block in iNKT cell development due to loss of NKAP is independent of Notch activation. The presence of iNKT cells in the thymus, liver and spleen from WT, CD4-cre NKAP cKO, CD4-cre RBP-Jκ cKO and CD4-cre NKAP cKO/ RBP-Jκ cKO mice were examined as in Fig. 1 . Data are representative of four independent experiments. Full size image iNKT cell development requires Hdac3 If the regulation of iNKT cell development by NKAP is independent of Notch activation, then NKAP must regulate additional pathways. We previously demonstrated that NKAP associates with Hdac3, and that transcriptional repression by NKAP requires its C-terminal DUF926 domain (domain of unknown function 926) that mediates binding to Hdac3 (ref. 8 ). If NKAP works together with Hdac3 to regulate iNKT cell development, then we would predict that thymocytes deficient in Hdac3 would phenocopy NKAP-deficient thymocytes and also exhibit a severe block in iNKT cell development. Although there was no gross alteration in conventional T-cell development in CD4-cre Hdac3 cKO mice, they also failed to generate iNKT cells, similar to CD4-cre NKAP cKO mice ( Fig. 7 ). Although Hdacs broadly regulate gene expression, the requirement of Hdac3 for iNKT but not conventional T cell development demonstrates that Hdac3 has unique functions in iNKT cells that cannot be compensated for by any other Hdac family member. The specificity of the defect for the iNKT cell lineage in the absence of either NKAP or Hdac3 indicates that these two associated proteins work together to regulate genes critical for this lineage. 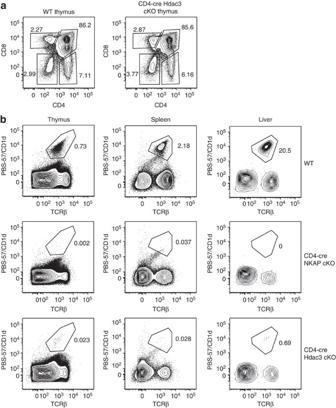Figure 7: Conditional deletion of Hdac3 also leads to a block in iNKT cell development. (a) DN, DP and SP thymocytes in WT and CD4-cre Hdac3 cKO mice were examined. Data shown are representative of four independent experiments. (b) The presence of iNKT cells in the thymus, liver and spleen from WT, CD4-cre NKAP cKO and CD4-cre Hdac3 cKO mice was examined as inFig. 1. Data are representative of four independent experiments. Figure 7: Conditional deletion of Hdac3 also leads to a block in iNKT cell development. ( a ) DN, DP and SP thymocytes in WT and CD4-cre Hdac3 cKO mice were examined. Data shown are representative of four independent experiments. ( b ) The presence of iNKT cells in the thymus, liver and spleen from WT, CD4-cre NKAP cKO and CD4-cre Hdac3 cKO mice was examined as in Fig. 1 . Data are representative of four independent experiments. Full size image We have demonstrated the absolute requirement for NKAP in the development of iNKT cells. iNKT cell development is blocked at the DP stage in CD4-cre NKAP cKO mice. Although there were small differences in expression of CD1d and SLAM family receptors in NKAP-deficient DP thymocytes compared with WT, the developmental defect in iNKT cells in CD4-cre NKAP cKO mice was cell-intrinsic as demonstrated by mixed bone marrow chimeras. The absence of iNKT cells in CD4-cre NKAP cKO mice was not due to decreased survival of thymocytes, as overexpression of a Bcl-xL or Bcl-2 transgene did not rescue iNKT cell development. There was no difference in the mRNA expression of anti-apoptotic Bcl-2 family genes Bcl-2 , Bcl-xL and Mcl-1 . Similar levels of Vα14-Jα18 rearrangement in genomic DNA from NKAP-deficient and WT DP thymocytes demonstrate that the defect in iNKT cell development is not due to an inability to rearrange the invariant TCRα chain. However, ectopic overexpression of the canonical Vα14-Jα18 TCR did restore iNKT cell development in CD4-cre NKAP cKO mice. Examination of genes that are required for iNKT cell development did not show changes in the expression of these genes resulting from NKAP deficiency, and the defect was also independent of Notch signalling. However, loss of the NKAP-associated protein histone deacetylase Hdac3 resulted in a similar lack of iNKT cells in the thymus, spleen and liver, suggesting that NKAP works with Hdac3 at an early stage in iNKT cell development. Therefore, NKAP controls entry of thymocytes into the iNKT cell lineage. To determine whether iNKT cell development in CD4-cre NKAP cKO mice could be rescued by a Vα14-Jα18 TCR transgene, a new line of mice had to be generated. Typically, TCR transgenes, even under the control of CD4 regulatory elements, are expressed prematurely at the DN stage [25] . This is a significant caveat to any examination of iNKT cell development using CD4-cre cKO mice, as the expression of the invariant TCR at the DN stage may permit positive selection into the iNKT cell lineage before cre-mediated deletion. Deleting NKAP earlier in development was not possible for these studies, as Lck-cre NKAP cKO mice have a severe defect in αβ T-cell development at the DN3 to DP transition, resulting in a 20-fold decrease in absolute DP thymocyte numbers [8] . Therefore, a new line of Vα14-Jα18 transgenic mice was generated, ‘rec-Vα14-Jα18’ in which Vα14-Jα18 is regulated by the endogenous TCRα LCR, using a modified pTα Cass transgene vector in which expression is dependent on RAG-mediated recombination, to replicate the endogenous pattern of expression for TCRα and prevent premature expression of the transgene [26] . However, this transgene is expressed at higher levels than the endogenous iNKT TCR, which may be due to use of Vα10 promoter in the transgenic construct rather than the endogenous Vα14 promoter. The increased expression of the transgenic recVα14-Jα18 TCR compensated for a defect in positive selection into lineage in NKAP-deficient DP thymocytes. However, we cannot exclude the possibility that the recVα14-Jα18 is expressed earlier in DP cell development, although it is not expressed at DN stage, than endogenously rearranged Vα14-Jα18 TCR, as the transgene uses optimized RSS sequences and is separated by only 5 kb, which may account for increased proportion of early-stage iNKT in recVα14-Jα18 mice. The role of NKAP in iNKT cell development is independent of its role as a negative regulator of Notch signalling, as abrogation of Notch-mediated activation through deletion of the transcription factor RBP-Jκ did not alleviate the block in iNKT cell development upon NKAP deletion. However, CD4-cre-mediated deletion of Hdac3, which associates with NKAP, resulted in the same phenotype as NKAP deletion, that is, loss of iNKT but not CD4 or CD8 SP cells. Although Hdacs broadly regulate gene expression, the specific requirement for Hdac3 for entry into the iNKT cell lineage demonstrates that Hdac3 has unique functions in iNKT cells that cannot be compensated for by any other Hdac family member. The specificity of the defect for the iNKT cell lineage in the absence of either NKAP or Hdac3 indicates that these two associated proteins work together to regulate genes critical for entry into the iNKT cell lineage. Interestingly, there is a complete block in iNKT cell development in CD4-cre Runx1 cKO mice, even though Vα14-Jα18 rearranges normally and is expressed equivalently at the mRNA level in Runx1-deficient DP thymocytes [6] . Runx1 has also been shown to associate with Hdac3 (ref. 30 ). Whether Runx1, Hdac3 and NKAP work together to regulate iNKT cell development is currently under investigation. Mice The generation of CD4-cre NKAP cKO mice was previously described [9] . RBP-Jκ floxed mice were generated and provided by T. Honjo (Kyoto University, Kyoto, Japan [29] ). Human Bcl-2 transgenic mice were generated by S. Korsmeyer (Dana-Farber Cancer Institute, Boston, MA [31] ) and provided by A. Singer (National Institutes of Health, Bethesda, MD). Bcl-xl [32] and ER-cre [33] trangenic mice were purchased from the Jackson Laboratories. CD4-cre mice [34] were purchased from Taconic through the National Institute of Allergy and Infectious Disease emerging models programme. Rag2 (T490A) mice have been previously described [23] . Hdac3 fl/fl mice have been previously described [35] . Construction of the Rec-Vα14 transgene mirrors that previously described for the generation of Rec-HY mice [26] . Briefly, the rearranged iNKT TCRα chain Vα14-Jα18 was cloned into the pTαCass transgenic vector with a complete TCRα LCR. The start codon from Vα14 was separated from the rest of the coding sequence by a 5-kb ‘stuffer’ fragment containing RSS recombination sequences, thus requiring Rag-mediated recombination for expression of the transgenic TCR. Rec-Vα14-Jα18 mice were generated by the transgenic facility at the Memorial Sloan-Kettering Cancer Center. Mice were housed in a barrier facility, and all experiments were performed under the guidelines and with the approval of the Mayo Clinic or Memorial Sloan-Kettering Cancer Center Institutional Animal Care and Use Committee. All animals were analysed between 8 and 16 weeks of age. All genetically altered mice were examined with either littermate or age-matched controls. Generation of radiation chimeras B6.SJL donors and recipients were purchased from National Cancer Institute Frederick, and radiation chimera generation was performed as previously described [9] . Flow cytometry Fluorescence-activated cell sorting analysis was performed on an LSRII flow cytometer (BD) and all experiments were analysed using Flow Jo (Tree Star). After size gating on FSC-A/SSC-A, doublet exclusion was done using both FSC-H/FSC-W and SSC-H/SSC-W. Dead cells were excluded from analysis by staining with 4',6-diamidino-2-phenylindole (DAPI). The following tetramers were obtained through the NIH Tetramer Facility: PE-conjugated CD1d tetramer, and PE-conjugated CD1d tetramer loaded with the glycolipid PBS-57 that is recognized by iNKT TCRs. All other reagents for flow cytometry were purchased from Becton Dickinson, eBioscience or Biolegend. Intracellular staining Thymocytes were stained for surface CD4 and CD8 before being fixed and permeabilized using Foxp3 fix:perm buffer kit (eBioscience) as per the manufacturer’s instructions. Cells were then stained for intracellular Bcl-2 and Nur77. Isolation of stage 0 iNKT cells All sorting was performed with a FACSAria (Becton Dickinson). To isolate stage 0 iNKT cells, thymocytes were stained with PE-labelled PBS-57-loaded CD1d tetramer. Cells were positively selected with anti-PE magnetic beads (Miltenyi Biotec) and ran through a separation column. Stage 0 iNKT cells were sorted based on PBS-57-CD1d + TCRβ + CD24 + NK1.1 − from positively selected cells. DP cells were sorted from thymocytes stained and gated with antibodies to CD4 and CD8. Quantitative PCR mRNA was isolated from sorted populations using an RNeasy kit (Qiagen). Complementary DNA from stage 0 iNKT cells was generated and amplified using an Ovation PicoSL WTA kit (NuGen). cDNA from DP thymocytes was generated using Superscript III (Invitrogen). Taqman probes (Applied Biosystems) for c-Myc, c-Myb, Runx1, Bcl-xL, Bcl-2, Nur77, Mcl-1 and 18S were used. All other targets were examined using SybrGreen, using previously published primers for Cβ, SAP [36] , Egr2 ( [37] ), Fyn [38] , TCR Cα [39] , CBFβ [40] , T-bet [41] , HEB [41] , HPRT [41] and glyceraldehyde 3-phosphate dehydrogenase [42] . For the canonical Vα14-Jα18, the following primers were used: Vα14: 5′-TCAAACAGGACACAGGCAAAGG-3′ Jα18: 5′-TCCCTAAGGCTGAACCTCTATC-3′ An ABI RT-PCR StepOne Plus System (Applied Biosystems) was used and relative expression was calculated with the 2-ΔΔCT method [43] . Genomic analysis of TCR rearrangement Genomic DNA was isolated from sorted DP thymocytes (Qiagen). DNA concentration was measured using a Nanodrop (Thermo Scientific). DNA was diluted so that either 99, 33 or 11 ng were used in each PCR reaction. The primers used to measure Vα14-Jα18 were the same as described above for use in qPCR. Glyceraldehyde 3-phosphate dehydrogenase primers were previously described [44] . PCR products were separated by agarose gel electrophoresis and visualized by ethidium bromide staining. 4-OHT induction of ER-cre NKAP cKO mice WT and ER-cre NKAP cKO mice were injected intraperitoneally with 250 μl of 20 mg ml −1 4-OHT (Sigma) dissolved in corn oil (Sigma) daily for 5 consecutive days. Mice were allowed to rest 1 day before analysis. How to cite this article: Thapa, P. et al. The transcriptional repressor NKAP is required for the development of iNKT cells. Nat. Commun. 4:1582 doi: 10.1038/ncomms2580 (2013).